Voltage-induced spreading and superspreading of liquids The ability to quickly spread a liquid across a surface and form a film is fundamental for a diverse range of technological processes, including printing, painting and spraying. Here we show that liquid dielectrophoresis or electrowetting can produce wetting on normally non-wetting surfaces, without needing modification of the surface topography or chemistry. Additionally, superspreading can be achieved without needing surfactants in the liquid. Here we use a modified Hoffman-de Gennes law to predict three distinct spreading regimes: exponential approach to an equilibrium shape, spreading to complete wetting obeying a Tanner’s law-type relationship and superspreading towards a complete wetting film. We demonstrate quantitative experimental agreement with these predictions using dielectrophoresis-induced spreading of stripes of 1,2 propylene glycol. Our findings show how the rate of spreading of a partial wetting system can be controlled using uniform and non-uniform electric fields and how to induce more rapid superspreading using voltage control. The rate of spreading of a small droplet of a viscous liquid on a solid surface is determined by the balance between interfacial and viscous forces. This physical process can be characterized by the dependence of the edge speed, v e , on the dynamic contact angle, θ ( t ), and often obeys the Hoffman-de Gennes law, v E θ (cos θ Y −cos θ ) θ ( θ 2 − θ Y 2 ), where cos θ Y =( γ SV − γ SL )/ γ LV gives the Young’s law contact angle, θ Y , and is determined by the three interfacial tensions γ ij ( [1] , [2] ). In the case of complete wetting ( θ Y =0 o ) of a surface by a small droplet of a non-volatile oil, the time dependence of the dynamic contact angle obeys a simple power law θ 1/( t + t 0 ) n , where t 0 is a constant and n =3/10 for a spherical cap droplet (Tanner’s law) and n =2/7 for a circular arc cross-section stripe of constant volume [3] , [4] . When a solid surface is rough or structured the balance between interfacial forces changes resulting in a change in equilibrium contact angle; a partial wetting surface can become completely wetting. It also changes the driving force for spreading so that a transition from a cubic law to a linear law occurs for the edge speed [5] . Thus, the rate of spreading can be controlled by topography, but such control is by surface design and so cannot easily be changed. One method of controlling the equilibrium contact angle is to use the contact area of an electrically conducting droplet as a contact on a conducting substrate, which has a thin electrically insulating layer. In this case, a capacitive system is created in which the charging of the solid–liquid interface induces wetting [6] , [7] . This electrowetting-on-dielectric effect with voltage control of the equilibrium contact angle has found application in droplet microfluidics [8] , [9] , liquid-lenses [10] , [11] and electronic paper [12] . It has also been used to induce morphological changes from a spherical cap droplet shape to a stripe droplet shape and to study dynamics of filaments wetting along open, rectangular microfluidic grooves [13] , [14] , and to increase maximum coating speeds by delaying air entrainment [15] . Recently, we showed that liquid dielectrophoresis using non-uniform electric fields, non-conducting liquids and without any need for direct electrical contact could be used to enhance the spreading of a droplet; so-called dielectrowetting [16] . In both electrowetting and dielectrowetting the change of surface free energy, Δ F , due to a small change in area, Δ A , at the contact line of a liquid with a contact angle θ , in the presence of a voltage, V , can be written as [7] , [16] , where the γ ij are the interfacial tensions and the precise form for λ depends upon whether the system involves an electrowetting or a dielectrowetting energy contribution. The equilibrium state is given by ΔF =0 and when V =0 this gives the Young’s law contact angle, θ Y , satisfying cos θ Y =( γ SV − γ SL )/ γ LV , assuming the liquid is intrinsically partially wetting and an equilibrium contact angle can be defined. The dependence of the equilibrium contact angle, θ e ( V ), on the voltage, V , can be written as, For the electrowetting case, α = ε 0 ε r /2 dγ LV is the ratio of capacitive energy per unit area to the liquid–vapor interfacial energy per unit area. In this case, the capacitive energy depends on the permittivity ε 0 ε r of the insulating dielectric solid, its thickness d , and the liquid’s surface tension γ LV ( [6] , [7] ). In the case of dielectrowetting, the ratio of interfacial liquid dielectric energy per unit area to the liquid–vapor interfacial energy per unit area predicts that α = ε 0 ( ε l −1)/2 δγ LV , which depends on the permittivity difference ε 0 ( ε l −1) between the dielectric liquid and air and the extent of the electric potential penetration depth, δ ( [16] ). In this paper, we formulate a macroscopic theory of voltage-induced dynamic wetting to find an analogue to the Hoffman-de Gennes law that is independent of the specific droplet geometry and which is valid when the excess free energy takes the form of equation (1), applicable to both electrowetting or dielectrowetting. Experimentally, we focus on voltage-induced wetting of stripes of the dielectric liquid 1,2 propylene glycol using liquid dielectrophoresis. The voltage modified Hoffman-de Gennes law is shown to quantitatively reproduce the experimentally observed time dependencies of the dynamic contact angle in the three spreading regimes: (i) an exponential approach to equilibrium contact angle with a rate constant τ −1 α θ e 7/2 ( V ) when V<<V Th ; (ii) a Tanner’s law-type −2/7th power law dependence at the voltage needed to induce complete wetting, V=V Th ; and (iii) a −2/3rd power law dependence in a voltage-induced superspreading regime when V >> V Th . A voltage-controlled analogue to the Hoffman-de Gennes law It is possible to view the α parameter in equation (2) as an experimentally determined one given by the threshold voltage, V Th , needed to induce complete wetting and a vanishing contact angle, that is, θ e ( V Th )=0 o . Defining allows equation (2) to be re-written as, In a similar manner to topography enhanced wetting, which has been shown to give topography driven spreading [5] , we expect both electrowetting and dielectrowetting to modify the dynamics of spreading, as well as the final equilibrium state. From equation (1), the rate of change of the energy per unit length of the contact line due to the unbalanced interfacial forces, including the energy contribution from the electric field, is, where v E is the edge speed and the time dependencies have been shown explicitly. In the de Gennes macroscopic approach, the viscous dissipation of energy per unit length of contact line is given by [2] , [4] , [17] , [18] , [19] , [20] , [21] , where η is the viscosity of the liquid and k ′ is a constant representing the viscous dissipation over the volume of fluid from some microscopic cutoff scale up to a hypothetical boundary within the droplet [2] , [21] . This approximation to the viscous dissipation is based on the lubrication approximation, assuming a parabolic velocity profile. Equating the rate of change in energy to the viscous dissipation gives, This formula is the electric field extended Hoffman-de Gennes equation [1] , [2] for the edge speed, v E , dynamic contact angle, θ ( t ), relationship including the effects of electrowetting or dielectrowetting. This macroscopic approach does not take into account additional dissipation processes associated with a precursor film advancing ahead of the macroscopic contact line when the spreading power, S = γ SV − γ SL −γ LV , is positive and the liquid is complete wetting, as discussed by, for example, de Gennes [2] , and Bonn et al. [21] Equation (6) predicts three distinct regimes according to V<<V Th , V ~ V Th and V>>V Th . In the case that the liquid is partial wetting and the applied voltage increases the wetting by only a small amount, that is, V<<V Th and θ e ( V )>0 o , the edge speed-dynamic contact angle relationship can be written as, where Δ θ ( t )= θ ( t )− θ e ( V ) is assumed to be small. For a small non-volatile droplet or stripe of liquid this predicts an exponential approach to the voltage-determined equilibrium contact angle. In the case that V ~ V Th , the Hoffman law, v E θ 3 , is obtained, In the case that V >> V Th , the edge speed becomes directly proportional to the dynamic contact angle, that is, Equations (8) and (9) are derived under the assumption that the dynamic contact angle is small. Thus, in a similar manner to topographic enhancement of the capillary drive for spreading to obtain a superspreading law, a voltage-induced superspreading should be achievable on what would be a partial wetting surface in the absence of a voltage. It also provides an alternative to the use of surfactants to both induce wetting of a surface that would not normally wet (that is, superwetting), and to increase the rate of spreading (that is, superspreading) on surfaces [20] , [21] , [22] , [23] , [24] , [25] , [26] , [27] . Voltage-induced spreading of dielectric liquid stripes To investigate whether the predicted voltage-induced spreading and superspreading regimes could be realized experimentally, we used a dielectrowetting configuration to modify the spreading of small droplets of 1,2 propylene glycol with a volume of 0.08±0.01 μl into stripes with fixed width. The experimental configuration uses interdigitated electrodes of linewidth 40 μm and gaps of 40 μm on glass and with a thin 0.85 μm capping layer of SU-8 photoresist with a hydrophobic treatment (see [16] and inset in Fig. 1 ). In all experiments, we used a 10-kHz sine wave voltage applied to the interdigitated electrodes to generate the non-uniform electric field extending vertically into the liquid. 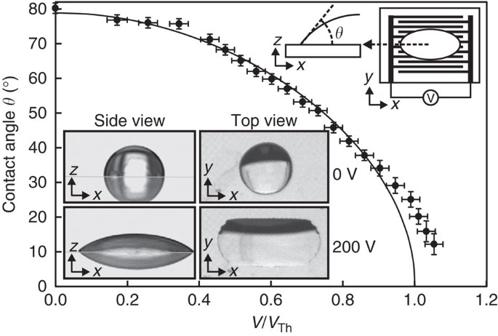Figure 1: Voltage-dependent equilibrium contact angles. The closed circles show the advancing equilibrium contact angle viewed perpendicular to the electrodes and measured in the long time limit with a constant amplitude sine wave voltage (10 kHz sine wave r.m.s.) applied to the electrodes. The solid line is a fit of equation (3) to the data below threshold; the deduced threshold voltage for inducing complete wetting isVTh=(230±2) V. Inset: schematic of experimental configuration, top view and side profile view (perpendicular to electrodes) of a droplet at 0 V and 200 V. Figure 1: Voltage-dependent equilibrium contact angles. The closed circles show the advancing equilibrium contact angle viewed perpendicular to the electrodes and measured in the long time limit with a constant amplitude sine wave voltage (10 kHz sine wave r.m.s.) applied to the electrodes. The solid line is a fit of equation (3) to the data below threshold; the deduced threshold voltage for inducing complete wetting is V Th =(230±2) V. Inset: schematic of experimental configuration, top view and side profile view (perpendicular to electrodes) of a droplet at 0 V and 200 V. Full size image We first determined the dependence of the equilibrium (long time limit) contact angle on the applied voltage by applying a droplet to the substrate with a constant amplitude voltage maintained during the spreading into a stripe, shown in Fig. 1 . The interdigitated electrode configuration provides a periodic energy barrier preventing spreading across the electrodes and so spreading progresses in the x -direction as a stripe configuration with the width of the liquid stripe in the y -direction remaining largely unchanged. Side and top view images of the resultant equilibrium droplet shape are shown inset in Fig. 1 for the example where 200 V was applied to the electrodes. The contact angle θ , defined in Fig. 1 , varies along the contour of the droplet shape in the y -direction at each advancing edge. Side view images of the equilibrium cross-sectional profile of droplets at each different voltage in the xz -plane were used to obtain the maximum contact angle at one advancing edge. The solid line in Fig. 1 is a fit of equation (3) to data below threshold, where the deduced threshold voltage for inducing complete wetting is V Th =(230±2) V. We then conducted a series of spreading experiments monitoring the dynamic contact angle θ and stripe width w in the x -direction with time for a fixed voltage; voltages below, near and above the threshold voltage were selected. In all of our experiments, the Weber number, which characterizes the relative importance of inertial and surface tension effects, satisfied W e <<1 and we have, therefore, neglected the effects of inertia in the analysis. 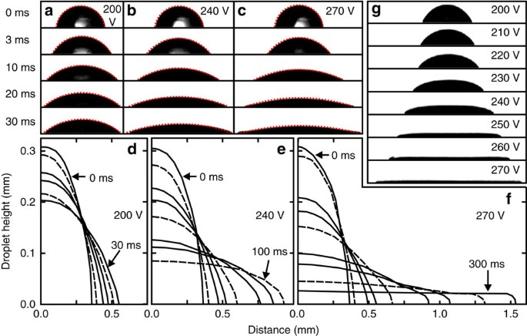Figure 2: Dynamic drop shape profiles at different spreading voltages. (a–c) show actual drop shape profiles viewed from they-direction and (d–f) show digitized drop shape profiles. The profiles are shown as a function of time after a constant amplitude sine wave voltage (10 kHz) is applied to the electrodes:aanddjust below the threshold voltage (200 V,V/VTh=0.87):bandejust above the threshold voltage (240 V,V/VTh=1.04); andcandffurther above the threshold voltage (270 V,V/VTh=1.17). In panelsd–fdigitized profiles are shown at times 0, 1 ms (dashed), 3 ms, 5 ms, 10 ms (dashed), 30 ms, 50 ms, 100 ms (dashed) and 300 ms. The red dashed lines shown ina–care fits to circular arcs. (g) Shows equilibrium (long time limit) droplet shapes viewed from they-direction for a range of different spreading voltages from 200 to 270 V. The vertical scale ingis expanded by a factor of 2 compared with the horizontal scale so that the spread film at 270 V can be clearly seen. Figure 2a–c show the profiles of droplets imaged from the y -direction during the dynamic spreading process at different instants in time, and at three different spreading voltages (200 V, 240 V and 270 V respectively). The droplet profiles were found to be very well described by circular arc sections, shown by the red dotted lines in Fig. 2 , for all times for spreading voltages of 200 V and below. As the voltage is increased significantly beyond 200 V the droplet profiles are circular arcs only for a restricted time after the onset of spreading, for example for times below 30 ms at 240 V, and for times below 20 ms at 270 V, as shown in Fig. 2b , respectively. For these higher voltages a transition to a film type cross-section at the foot of the profile can be observed at longer times. Digitized droplet profiles are shown in Fig. 2d–f for three different spreading voltages (200 V, 240 V and 270 V, respectively) covering a full range of times from the start of spreading to when the droplet shape is close to equilibrium. This illustrates the distinct non-circular profile at 270 V for which the contact angle at the advancing edge is not as well defined. Images of the evolution of the equilibrium (long time limit) shape of the droplet with voltage at high voltages are shown in Fig. 2g . Figure 2: Dynamic drop shape profiles at different spreading voltages. ( a – c ) show actual drop shape profiles viewed from the y -direction and ( d – f ) show digitized drop shape profiles. The profiles are shown as a function of time after a constant amplitude sine wave voltage (10 kHz) is applied to the electrodes: a and d just below the threshold voltage (200 V, V / V Th =0.87): b and e just above the threshold voltage (240 V, V / V Th =1.04); and c and f further above the threshold voltage (270 V, V / V Th =1.17). In panels d – f digitized profiles are shown at times 0, 1 ms (dashed), 3 ms, 5 ms, 10 ms (dashed), 30 ms, 50 ms, 100 ms (dashed) and 300 ms. The red dashed lines shown in a – c are fits to circular arcs. ( g ) Shows equilibrium (long time limit) droplet shapes viewed from the y -direction for a range of different spreading voltages from 200 to 270 V. The vertical scale in g is expanded by a factor of 2 compared with the horizontal scale so that the spread film at 270 V can be clearly seen. Full size image To analyse the data, we applied the conservation of volume of the liquid, Ω, and the circular arc cross-section stripe geometry for a stripe of length L 0 in the y -direction. The assumption is that the spreading alters the circular arc defined by the contact angle, θ (assumed small) and contact width on the substrate, w =2 x 0 , but always conserves the volume of liquid. From geometry, the edge speed of the contact line on the substrate is given by McHale et al . [4] , Thus, to first order in the prefactor, the electric field extended form of the Hoffman-de Gennes law, equation (6), for a circular arc cross-section stripe of constant volume can be written as, where α = k ( γ LV / η )(8 L 0 /3Ω) 1/2 . The assumption that the prefactor can be expanded is numerically reasonable for contact angles below around 60 o because the series only involves even powers. Equation (12) allows solutions to be obtained for the dynamic contact angle behaviour with time in each of the three regimes V<<V Th , V ~ V Th and V >> V Th . In the case that V << V Th , the dynamic contact angle is predicted to approach its long time limit equilibrium value, θ e , exponentially, that is, where τ −1 = k ( γ LV / η )(8 L 0 /3Ω) 1/2 θ e 7/2 ( V ) and Δ θ 0 = θ ( t =0)− θ e is the constant of integration. 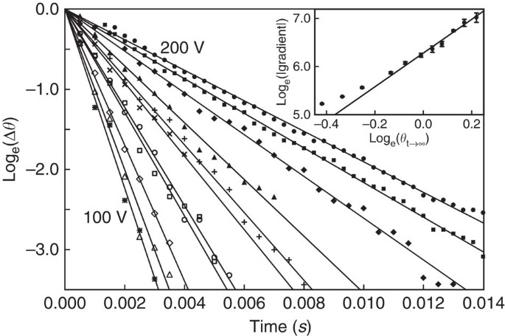Figure 3: Exponential approach to equilibrium of spreading stripes on interdigital electrodes. The applied voltages are below the threshold voltage. For clarity, all curves have been offset to pass through the origin. Δθis the difference between the dynamic contact angle and the equilibrium contact angle at a particular voltage. Data are shown for applied voltages at 10 V intervals between 100 V (asterisks) and 200 V (filled circles). Inset: Test of the predicted dependenceθe(V)−7/2for the time constant in the exponential approach to equilibrium; the solid line has a slope of 7/2. Figure 3 shows the dependence of log e (Δ θ ) with time for the spreading of stripes for voltages in 10 V steps from 100 to 200 V so that all are below the threshold voltage. The solid lines are linear regression fits to the data. According to equation (13) these slopes should reduce as the voltage is increased and the wetting becomes stronger. The inset to Fig. 3 tests quantitatively whether the time constant in the approach to equilibrium follows a θ e ( V ) −7/2 power law as predicted by equation (13). This shows that for voltages away from the threshold, the exponential approach is well-described by equation (13) but, as expected, the data is less well-described by this equation as V → V Th . Figure 3: Exponential approach to equilibrium of spreading stripes on interdigital electrodes. The applied voltages are below the threshold voltage. For clarity, all curves have been offset to pass through the origin. Δ θ is the difference between the dynamic contact angle and the equilibrium contact angle at a particular voltage. Data are shown for applied voltages at 10 V intervals between 100 V (asterisks) and 200 V (filled circles). Inset: Test of the predicted dependence θ e ( V ) −7/2 for the time constant in the exponential approach to equilibrium; the solid line has a slope of 7/2. Full size image In the case that V ~ V Th , the dynamic contact angle tends to zero in the long time limit, and integration of equation (12) gives, where t 0 is a constant of integration. The dynamic contact angle is predicted to decrease according to a −2/7th power law in time as previously reported for the complete wetting of stripes of polydimethylsiloxane on glass slides. This is the stripe form of Tanner’s law, which holds for complete spreading of axisymmetric droplets of polydimethylsiloxane [4] . In the case that V>>V Th , integration of equation (12) gives, where t 0 is a constant of integration. The dynamic contact angle is predicted to follow a −2/3rd power law in time. The clear linear dependences shown in Fig. 4 confirm that the power law relationship, θ 1/( t + t 0 ) n , holds for voltages between 200 V and 270 V, where the value of n is given by the gradient at each voltage. The inset in Fig. 4 show the value of the exponent n rises from close to 2/7 at voltages just below V Th to 2/3 as the voltage is increased above V Th , in excellent agreement with the predictions of equations (14) and (15). 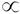Figure 4: Power law spreading and superspreading of stripes on interdigital electrodes showing dynamic contact angleθ1/(t+t0)n. Data are shown for applied voltages of 200 V (filled circle), 210 V (filled square), 220 V (filled diamond), 230 V (filled triangle), 235 V (plus), 240 V (cross), 255 V (open circle), 265 V (open square) and 270 V (open diamond). The time is denoted byt, andt0is a constant at each voltage. For clarity, all curves have been offset to pass through the origin. Inset:nis close to 2/7 at voltages just belowVTh, rising to 2/3 as the voltage is increased aboveVTh. Figure 4: Power law spreading and superspreading of stripes on interdigital electrodes showing dynamic contact angle θ 1/( t + t 0 ) n . Data are shown for applied voltages of 200 V (filled circle), 210 V (filled square), 220 V (filled diamond), 230 V (filled triangle), 235 V (plus), 240 V (cross), 255 V (open circle), 265 V (open square) and 270 V (open diamond). The time is denoted by t , and t 0 is a constant at each voltage. For clarity, all curves have been offset to pass through the origin. Inset: n is close to 2/7 at voltages just below V Th , rising to 2/3 as the voltage is increased above V Th . Full size image Using the relationship v e ( t )= 1 / 2 ( dw ( t )/ dt ), equation (12), and the dynamic contact angle expressions, also allows solutions to be obtained for the dynamic contact width, w ( t ), behaviour with time. These are given in equations (16), (17) and (18) for each of the three regimes V << V Th , V ~ V Th and V >> V Th , respectively, Below the threshold voltage V / V Th <1, the dynamic contact width tends to a constant value, w e =2 x e , in the long time limit and so equation (16) is written in terms of the difference from the equilibrium contact half-width, Δ x ( t )= x 0 ( t )− x e . In this regime, the contact width approaches its equilibrium value exponentially with the same time constant as that for the exponential approach to equilibrium of the contact angle. The clear linear dependences shown in Fig. 5 confirm that the power law relationship, w 1/( t + t 0 ) n , also holds for the stripe width for voltages between 200 and 270 V where the value of n is given by the gradient at each voltage. The inset in Fig. 5 shows that the classic Tanner spreading law for a stripe in equation (17), w ~( t + t 0 ) 1/7 , is found at 200 V and a superspreading regime is found at higher voltages in which the magnitude of the spreading exponent increases as the voltage is increased, reaching w ~( t + t 0 ) 1/3.39 at 270 V; this is consistent with the theoretically expected power law in equation (18) of w ~( t + t 0 ) 1/3 . The increase in this exponent is a characteristic of ‘superspreading’ phenomenon referred to in [25] and other references on superspreading achieved through surfactants. These data illustrate that partial wetting systems can be forced to become wetting and that a transition to a more rapid superspreading regime can be achieved in a relatively simple manner. 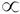Figure 5: Power law spreading and superspreading of stripes on interdigital electrodes showing dynamic contact widthw1/(t+t0)n. Data are shown for applied voltages of 200 V (filled circle), 220 V (filled diamond), 230 V (filled triangle), 250 V (open circle), and 270 V (open diamond). The time is denoted byt, andt0is a constant at each voltage. Inset:nis close to 1/7 at voltages just belowVTh, the classic ‘Tanner’ spreading law for a stripe, rising to 1/3.39 as the voltage is increased significantly aboveVTh. Figure 5: Power law spreading and superspreading of stripes on interdigital electrodes showing dynamic contact width w 1/( t + t 0 ) n . Data are shown for applied voltages of 200 V (filled circle), 220 V (filled diamond), 230 V (filled triangle), 250 V (open circle), and 270 V (open diamond). The time is denoted by t , and t 0 is a constant at each voltage. Inset: n is close to 1/7 at voltages just below V Th , the classic ‘Tanner’ spreading law for a stripe, rising to 1/3.39 as the voltage is increased significantly above V Th . Full size image In this work, we have formulated a macroscopic theory of voltage-induced dynamic wetting that extends the Hoffman-de Gennes law and which is independent of the specific droplet geometry. Experimentally, we have focused on stripes of a dielectric liquid using liquid dielectrophoresis to achieve the voltage control. However, the same principles apply to axisymmetric ‘spherical cap’ droplets and in this case three regimes are also predicted, giving a dynamic contact angle with: an exponential approach to equilibrium contact angle with a rate constant τ −1 = k ( γ LV / η )(27 π /4Ω) 1/3 θ e 10/3 ( V ) when V << V Th ,; a −3/10th power law at complete wetting when V ~ V Th ; and a −3/4 power law in the voltage-induced superspreading regime when V >> V Th ( Supplementary Equations (S3), (S4) and (S5) in Supplementary Note 1 ). The cross-over from an exponent of −3/10 to −3/4 is the same as for topography-induced superspreading [5] , but with voltage rather than roughness controlling the transition and its strength. The corresponding behaviour for the axisymmetric droplet contact radius is an exponential approach to equilibrium with the same rate constant as for the contact angle, a 1/10th power law at complete wetting, and ¼ power law in the voltage-induced superspreading regime ( Supplementary Equations (S6), (S7) and (S8) in Supplementary Note 1 ). This can be compared with the exponents measured for surfactant-induced superspreading of axisymmetric droplets, which have been reported to increase from the 1/10th power law up to as much as a linear law with time depending on concentration of surfactant [21] , [26] . In our experiments, we have used liquid dielectrophoresis as the controlling method, but the theory and formulae apply equally to voltage control achieved using an electrowetting configuration. Our theory and measurements show that it is possible to induce spreading on an otherwise partially wetting substrate using electric fields. This is an approach complementary to the use of topographic or chemical modification of the solid surface or modification of the liquid by including surfactants or otherwise. It has the advantage that the final equilibrium contact angle or the strength of the superspreading can be tuned simply by adjusting an applied voltage. This work has relevance for any process involving control of films, such as in inking and painting where controlled spreading of droplets may be beneficial [28] , or in high speed coating involving forced wetting where increasing the wetting delays the onset of bubble entrainment [15] , [29] . Device fabrication The device substrate was a borosilicate glass slide of thickness 1.1 mm, which was precoated with a 25-nm layer of indium tin oxide of resistivity 100 Ohm per square (Praezisions Glas and Optik GmbH, Iserlohn, Germany). The experimental configuration used interdigitated electrodes of linewidth 40 μm and gaps of 40 μm on glass covering an area of 5 mm by 5 mm. The indium tin oxide electrodes were patterned using standard photolithographic procedures using S1813 photoresist (Shipley Europe Ltd, Coventry, UK). The pattern was etched in a solution of 12.5% 1 M hydrochloric and 12.5% 1 M nitric acid in water for 6 min. A thin 0.85 μm capping layer of SU-8 negative photoresist (MicroChem Corp., Newton, MA, USA) on top of the electrodes was used to help prevent electrical breakdown. This was produced by spinning 30:70 by volume of SU-8 10 negative photoresist and Microposit EC solvent (ROHM and HAAS Europe trading APS, Lyngby, Denmark) onto the substrates (10 s at 500 r.p.m. and 30 s at 3,000 r.p.m. ), followed by soft baking (65 °C for 1 min, then 95 °C for 1 min), flood ultraviolet exposure (6 s in a Microtec SUSS MJ4B Mask Aligner) and hard baking (65 °C for 1 min, then 95 °C for 3 min, then 155 °C for 10 min). An ultraviolet/ozone treatment and a hydrophobic treatment were applied to the SU-8 capping layer. This treatment increases the contact angle of sessile droplets of 1,2 propylene glycol on the surface. The SU-8 samples were oxidized in a UV/Ozone ProCleaner (Bioforce Nanoscience Inc., Ames, IA, USA) for 20 min, then immersed in Granger’s solution (Granger’s Extreme Wash-in, Grangers International Ltd, Alfreton, Derbyshire UK) diluted to 1:20 by volume in deionised water for 20 min, followed by rinsing in deionised water, drying with nitrogen gas and baking at 80 °C for 20 min. Actuation of voltage-induced spreading A volume-calibrated ‘Gilson Pipetman’ micropipette (Gilson, Inc., Middleton, USA) was used to dispense 1,2 propylene glycol droplet into the centre of the electrode area. Droplet volumes used were in the range 0.08±0.01 μl. Electrical addressing of the device was performed with a 10-kHz sine wave voltage provided by a TTi TGA1244 arbitrary wave form generator (Thurlby Thander Instruments Limited, Cambs, UK) connected to a PZD700A-1 amplifier (Trek Inc., Medina, New York, USA). The voltage was applied to each alternate electrode finger with the interposed electrodes at earth potential. All voltages reported are root mean square values. Measurement of dynamic contact angles The measurement geometry is shown inset in Fig. 1 . Time dependent side view images of the droplet during voltage spreading were obtained from the y -direction (side view) using a high speed video camera (Hotspot, NAC Image Techonology, Devon, UK) fitted with a × 10 objective lens, while the top view from the z -direction was monitored using a standard USB video camera (DCC1645C, ThorLabs, Ely, UK) fitted with a × 4 objective lens. The dynamic contact angles were obtained from the greyscale images of the droplet taken from the y -direction ( Fig. 1 ) during voltage spreading analysed using automated Drop Shape Analysis software (KRÜSS GmbH, Hamburg, Germany). The images were contrast enhanced to make the edges of the droplet distinct using a mapping with three linear sections between (0,0), (76,0), (181,255) and (255,255), where the first number in the brackets is the input pixel greylevel and the second is the output pixel greylevel. The baseline was defined manually, and this did not change for a sequence of images at a given voltage. The Drop Shape Analysis software fitted a circular arc to each image in the sequence and then extracted the contact angle values used in Figs 1 , 3 and 4 from the height and width of the arc using standard trigonometry. An exception applied to the equilibrium contact angle values obtained for voltages between 210 and 245 V in Fig. 1 : the droplet profiles at these voltages, shown in Fig. 2g , were not well-described by circular arcs and so these contact angles were calculated manually from the gradient at the advancing edge of the droplet. How to cite this article: McHale, G. et al. Voltage-induced spreading and superspreading of liquids. Nat. Commun. 4:1605 doi: 10.1038/ncomms2619 (2013).